Natural variation in arsenate tolerance identifies an arsenate reductase inArabidopsis thaliana The enormous amount of environmental arsenic was a major factor in determining the biochemistry of incipient life forms early in the Earth’s history. The most abundant chemical form in the reducing atmosphere was arsenite, which forced organisms to evolve strategies to manage this chemical species. Following the great oxygenation event, arsenite oxidized to arsenate and the action of arsenate reductases became a central survival requirement. The identity of a biologically relevant arsenate reductase in plants nonetheless continues to be debated. Here we identify a quantitative trait locus that encodes a novel arsenate reductase critical for arsenic tolerance in plants. Functional analyses indicate that several non-additive polymorphisms affect protein structure and account for the natural variation in arsenate reductase activity in Arabidopsis thaliana accessions. This study shows that arsenate reductases are an essential component for natural plant variation in As(V) tolerance. Groundwater contamination with arsenic is a threat for most organisms, including man [1] , [2] , [3] . In plants, arsenic tolerance is critical for adaptation to specific soils and has determined plant distribution [4] , [5] ; the molecular mechanisms are analyzed mainly by studying proteins presumably involved in arsenate (As(V)) tolerance based on sequence homology with bacterial and yeast proteins [6] , [7] . Genetic approaches are little used to study As(V) tolerance mechanisms [8] , [9] , [10] , [11] , [12] , and the genes implicated in natural intraspecific variation are unknown [13] , [14] , [15] . Here we address the natural genetic variation of Arabidopsis thaliana for arsenate tolerance, leading to the identification of a major effect quantitative trait locus (QTL) ATQ1 . Molecular isolation and characterization of this locus showed that it encodes a novel plant arsenate reductase whose contribution to the natural variation for arsenate tolerance is caused by several functional polymorphisms. Natural variation identifies a QTL for arsenate tolerance We evaluated variation in As(V) tolerance in a collection of 82 A. thaliana accessions with a broad geographic distribution ( Supplementary Data 1 ). Using a root growth recovery (RGR) assay, we quantified the percentage of plants that recovered root growth in As(V)-free medium after brief As(V) exposure ( Supplementary Fig. 1a ). We found substantial genetic variation among accessions, which defines two phenotypic groups for As(V) tolerance ( Fig. 1a ). The first, with a clear As(V)-sensitive phenotype, is represented by genotype Kashmir-1 (Kas-1; 7% RGR), and the other is comprised of accessions with As(V) tolerance similar to that of Col gl -1 (Col) in which 77% of plants recovered root growth after As(V) exposure ( Fig. 1a,b ). As(V) tolerance can be associated with slow As(V) uptake [11] , [16] , [17] and correlates with enhanced arsenic accumulation [8] , [11] . We observed that Col accumulated three times more arsenic than Kas-1 ( Supplementary Fig. 1b ); nonetheless, both accessions show similar As(V) uptake ( Supplementary Fig. 1c ), suggesting that other mechanisms may be responsible for this strong phenotypic variation. 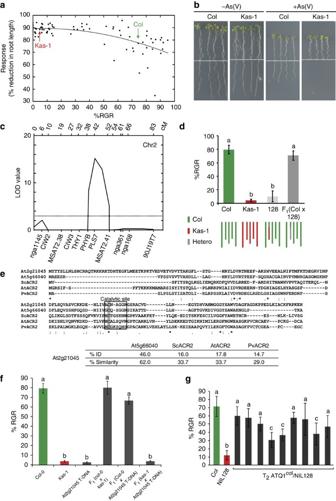Figure 1: Identification ofATQ1for As(V) tolerance. (a) Quantification of As(V) tolerance phenotype in 82 Arabidopsis accessions. The percentage of root growth reduction in response to 15 μM As(V) is plotted against the percentage of plants that recover root growth after 24 h exposure to 15 μM As(V) (%RGR; see Methods). Colgl-1(Col; green) and Kashmir (Kas-1; red) are indicated. (b) As(V) tolerance phenotype of Colgl-1(Col) and Kashmir (Kas-1) plants using the RGR assay. Dotted line indicates starting point of root growth in +Pi medium. (c) LOD score values from multiple QTL mapping analysis.ATQ1mapping is shown between markers PHYB and MSAT2.41. (d) Confirmation ofATQ1. NIL128 and Col x NIL128 F1plants were used for %RGR determination. Graphical genotypes are shown beneath the graph. Bars show mean±s.d. (n=3). (e) Alignment of Col-0 AT2G21045 protein with theArabidopsis thalianasulfurtransferase (AT5G66040) and with arsenate reductases fromSaccharomyces cerevisiaeScACR2 (NP_015526),Arabidopsis thalianaAtACR2 (AT5G03455) andPteris vittataPvACR2 (ADP20951). The catalytic site with the active cysteine residue (grey background) is shown (box). ‘*’ (asterisk) indicates positions with a single, fully conserved residue, ‘:’ (colon) and a ‘.’ (period) indicate conservation of amino acids with strong and weak similarity in properties, respectively. The table shows percentages of amino acid sequence identity (%ID) and similarity between AT2G21045 and other proteins in the alignment. (f,g) Quantitative complementation test forATQ1. (f) Col-0, Kas-1, At2g21045 T-DNA, the F1from crosses of Col-0 or Kas-1 with At2g21045 T-DNA plants and (g) Colgl-1(Col), NIL128 and the T2of nine independent At2g21045-overexpressing lines (T2ATQ1Col/NIL128) were used for %RGR determination. Bars show mean±s.d. (n=3). Means with different letters are significantly different (t-test,P<0.05). Figure 1: Identification of ATQ1 for As(V) tolerance. ( a ) Quantification of As(V) tolerance phenotype in 82 Arabidopsis accessions. The percentage of root growth reduction in response to 15 μM As(V) is plotted against the percentage of plants that recover root growth after 24 h exposure to 15 μM As(V) (%RGR; see Methods). Col gl-1 (Col; green) and Kashmir (Kas-1; red) are indicated. ( b ) As(V) tolerance phenotype of Col gl-1 (Col) and Kashmir (Kas-1) plants using the RGR assay. Dotted line indicates starting point of root growth in +Pi medium. ( c ) LOD score values from multiple QTL mapping analysis. ATQ1 mapping is shown between markers PHYB and MSAT2.41. ( d ) Confirmation of ATQ1 . NIL128 and Col x NIL128 F 1 plants were used for %RGR determination. Graphical genotypes are shown beneath the graph. Bars show mean±s.d. ( n =3). ( e ) Alignment of Col-0 AT2G21045 protein with the Arabidopsis thaliana sulfurtransferase (AT5G66040) and with arsenate reductases from Saccharomyces cerevisiae ScACR2 (NP_015526), Arabidopsis thaliana AtACR2 (AT5G03455) and Pteris vittata PvACR2 (ADP20951). The catalytic site with the active cysteine residue (grey background) is shown (box). ‘*’ (asterisk) indicates positions with a single, fully conserved residue, ‘:’ (colon) and a ‘.’ (period) indicate conservation of amino acids with strong and weak similarity in properties, respectively. The table shows percentages of amino acid sequence identity (%ID) and similarity between AT2G21045 and other proteins in the alignment. ( f , g ) Quantitative complementation test for ATQ1 . ( f ) Col-0, Kas-1, At2g21045 T-DNA, the F 1 from crosses of Col-0 or Kas-1 with At2g21045 T-DNA plants and ( g ) Col gl-1 (Col), NIL128 and the T 2 of nine independent At2g21045-overexpressing lines (T 2 ATQ1 Col /NIL128) were used for %RGR determination. Bars show mean±s.d. ( n =3). Means with different letters are significantly different ( t -test, P <0.05). Full size image To determine the genetic basis of natural variation for As(V) tolerance in A. thaliana, we used QTL mapping for the RGR trait in a Col x Kas-1 recombinant inbred line (RIL) population [18] . We found a large effect locus that accounts for 55% of the phenotypic variance on chromosome 2 ( Fig. 1c , Supplementary Data 2 ), which we termed arsenate tolerance QTL1 ( ATQ1 ). The ATQ1 effect was confirmed in near-isogenic lines (NIL) derived from a specific ATQ1- Kas-1 RIL ( Supplementary Fig. 1d ). NIL bearing ATQ1 -Kas-1 alleles introgressed in the Col background showed a percentage of RGR similar to that of Kas-1 parental plants ( Supplementary Fig. 1d ), and F 1 plants derived from the NIL128 x Col cross behaved similarly to Col parents; these data indicate that the As(V)-sensitive allele ATQ1 -Kas-1 is recessive ( Fig. 1d ). QTL mapping for As(V) tolerance in a RIL population derived from As(V)-sensitive Tsu-0 and the Col-0 reference strain also detected a major effect QTL in the same genetic position ( Supplementary Fig. 2 , Supplementary Data 3 ). The similar effect and location of the Tsu-0 x Col-0 QTL and ATQ1 suggested that this is the main locus responsible for natural A. thaliana variation in As(V) tolerance. ATQ1 encodes a rhodanase-like protein ATQ1 was fine-mapped using an F 2 population of 679 plants derived from the NIL128 × Col cross ( Supplementary Fig. 3 ). Phenotypic characterization of selected F 3 /F 4 homozygous recombinants located ATQ1 in a 0.7-Mb genomic region between positions 8.9 and 9.6 Mb ( Supplementary Fig. 3 ). Further analysis of this region for ATQ1 candidate genes identified At2g21045 as a gene encoding a protein with 46% identity and 62% similarity with the At5g66040 sulphur transferase of the rhodanase family [19] ( Fig. 1e ). The presence of a rhodanase domain is characteristic of eukaryotic As(V) reductases [19] , [20] , [21] , an activity which might be responsible for arsenate tolerance. To test whether At2g21045 is responsible for ATQ1 , we characterized a transfer DNA (T-DNA) insertion mutant of this gene in the Col-0 background, As(V) sensitivity was similar to that of Kas-1 plants ( Fig. 1f ). In phenotypic analyses of F 1 plants derived from a cross between the At2g21045 T-DNA mutant and Kas-1, the ATQ1 -Kas-1 allele did not complement the mutant phenotype for the RGR trait ( Fig. 1f ). The As(V)-tolerant phenotype of transgenic plants that overexpressed At2g21045-Col gene in a NIL128 background resembled that of the parental Col accession ( Fig. 1g ). These results indicated that the At2g21045 gene is ATQ1, whose Col and Kas-1 alleles account for natural variation in As(V) tolerance. ATQ1 reveals a new arsenate reductase To identify the underlying molecular mechanism, we tested whether ATQ1 /At2g21045 encoded an As(V) reductase. Structural modelling analyses of ATQ1/AT2G21045 protein suggested that it retains the overall rhodanase fold characteristic of As(V) reductases ( Supplementary Fig. 4a,b ). Col plants exposed to trinitrobenzenesulphonic acid (TNBS, a rhodanase inhibitor) showed an As(V)-sensitive phenotype. Although TNBS has an effect on thiol content [22] , this observation suggests that a rhodanase-like protein might be responsible for As(V) tolerance in Col accession ( Supplementary Fig. 4c ). The ATQ1/AT2G21045 sequence has a cysteine residue (Cys 113 in Col-0; Fig. 1e ) in a C(X) 4 R motif similar to C(X) 3 R or HC(X) 5 R, characteristic of the As(V) reductase catalytic active site [21] , [23] . Increased sensitivity to As(V) but not to As(III) is a characteristic of As(V) reductase mutants [24] . Analyses of As(V) and As(III) tolerance showed that Kas-1, NIL128 and the ATQ1/At2g21045 T-DNA mutant were highly sensitive to As(V) but not to As(III) compared with Col-0 plants, further supporting that ATQ1 encodes an arsenate reductase ( Fig. 2a,b ). 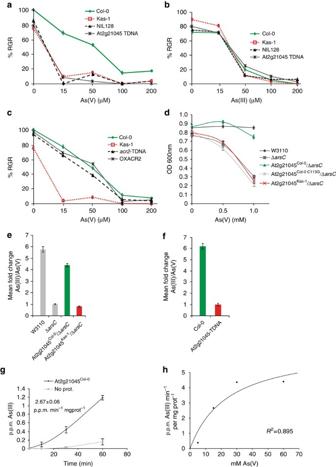Figure 2: Arabidopsis At2g21045 gene encodes an arsenate reductase. (a) As(V) and (b) As(III) tolerance analysis of Col-0, Kas-1, NIL128 and the At2g21045 T-DNA mutant. Percentage of RGR (%RGR) was determined at various As(V) and As(III) concentrations. Bars show mean±s.d. (n=3). (c)Atacr2T-DNA mutant (acr2-T-DNA) and ACR2-overexpressing lines (OXACR2) have an As(V) tolerance phenotype similar to that of Col-0. %RGR was determined at various As(V) concentrations. Bars show mean±s.d. (n=3). (d) Complementation analysis ofE. coliΔarsCstrain. Wild-type strain W3110, WC3110 with anarsCgene deletion (ΔarsC), ΔarsCexpressing the At2g21045-Col-0 allele (At2g21045Col-0/ΔarsC) or expressing this allele with replacement of the active Cys113by Gly113(At2g21045ColC113G/ΔarsC) or expressing the At2g21045 Kas-1 allele (At2g21045Kas-1/ΔarsC) were grown in various As(V) concentrations. Values are mean±s.d. (n=3). (e) Arsenic species analysis in culture supernatants ofE. coliwild type (W3110), ΔarsC, ΔarsCexpressing the At2g21045-Col-0 allele (At2g21045Col-0/ΔarsC) or ΔarsCexpressing the At2g21045 Kas-1 allele (At2g21045Kas-1/ΔarsC) exposed to As(V) 24 h. Bars show mean±s.d. (n=3). (f) Arsenic species analysis of extracts of Col-0 and At2g21045 T-DNA mutant plants exposed to 5 μM As(V; 24 h). Values are mean±s.d. (n=5). (g,h)In vitroAT2G21045 arsenate reductase activity. (g) Arsenate reductase activity measured as As(III) production of a recombinant AT2G21045 protein in the presence of 15 mM As(V). Same analysis was conducted in the absence of protein (No Prot). Graph represents parts per million (p.p.m.) of As (III). The value of the specific enzymatic activity is given. Data shows mean±s.d. (n=3). (h) Arsenate reductase activity of recombinant AT2G21045 protein with increasing As(V) concentrations. AKmvalue of 25 was estimated using SigmaPlot v.12.5 for non-linear regression analysis. The coefficient of determination (R2) used to fit the data to a curve is given. Figure 2: Arabidopsis At2g21045 gene encodes an arsenate reductase. ( a ) As(V) and ( b ) As(III) tolerance analysis of Col-0, Kas-1, NIL128 and the At2g21045 T-DNA mutant. Percentage of RGR (%RGR) was determined at various As(V) and As(III) concentrations. Bars show mean±s.d. ( n =3). ( c ) Atacr2 T-DNA mutant ( acr2 -T-DNA) and ACR2-overexpressing lines (OXACR2) have an As(V) tolerance phenotype similar to that of Col-0. %RGR was determined at various As(V) concentrations. Bars show mean±s.d. ( n =3). ( d ) Complementation analysis of E. coli Δ arsC strain. Wild-type strain W3110, WC3110 with an arsC gene deletion (Δ arsC ), Δ arsC expressing the At2g21045-Col-0 allele (At2g21045 Col-0 /Δ arsC ) or expressing this allele with replacement of the active Cys 113 by Gly 113 (At2g21045 ColC113G /Δ arsC ) or expressing the At2g21045 Kas-1 allele (At2g21045 Kas-1 /Δ arsC ) were grown in various As(V) concentrations. Values are mean±s.d. ( n =3). ( e ) Arsenic species analysis in culture supernatants of E. coli wild type (W3110), Δ arsC , Δ arsC expressing the At2g21045-Col-0 allele (At2g21045 Col-0 /Δ arsC ) or Δ arsC expressing the At2g21045 Kas-1 allele (At2g21045 Kas-1 /Δ arsC ) exposed to As(V) 24 h. Bars show mean±s.d. ( n =3). ( f ) Arsenic species analysis of extracts of Col-0 and At2g21045 T-DNA mutant plants exposed to 5 μM As(V; 24 h). Values are mean±s.d. ( n =5). ( g , h ) In vitro AT2G21045 arsenate reductase activity. ( g ) Arsenate reductase activity measured as As(III) production of a recombinant AT2G21045 protein in the presence of 15 mM As(V). Same analysis was conducted in the absence of protein (No Prot). Graph represents parts per million (p.p.m.) of As (III). The value of the specific enzymatic activity is given. Data shows mean±s.d. ( n =3). ( h ) Arsenate reductase activity of recombinant AT2G21045 protein with increasing As(V) concentrations. A K m value of 25 was estimated using SigmaPlot v.12.5 for non-linear regression analysis. The coefficient of determination ( R 2 ) used to fit the data to a curve is given. Full size image In A. thaliana it has been previously described that another rhodanase protein, AtACR2, homologue to the yeast arsenate reductase, is able to complement the E. coli arsenate reductase mutant suggesting that AtACR2 encodes an As(V) reductase ( Fig. 1e ). In contrast, using our RGR system we found no differences in As(V) sensitivity in Atacr2 T-DNA knockout or ACR2 -overexpressing lines compared with Col-0 ( Fig. 2c ). Although the biological significance of AtACR2 was questioned in a study [25] , Atacr2 knockout line showed no arsenate reductase activity [26] but displayed a remarkable As(V)-sensitive phenotype [25] , [27] . Therefore we cannot exclude the possibility that under certain conditions AtACR2 has a relevant role in As(V) tolerance as an As(V) reductase. Phylogenetic analysis shows that ATQ1/AT2G21045 is remarkably different from the ACR2 rhodanase clade ( Supplementary Fig. 5 ). In fact, the large diversity of the widespread protein rhodanase family does not allow the identification of a conserved AT2G21045 ortholog in most plant species further than A. thaliana closest relatives. We thus concluded that At2g21045 encodes a new rhodanase protein responsible for the natural genetic variability for arsenate tolerance in A. thaliana . To determine whether At2g21045 encodes a bona fide As(V) reductase, we used functional complementation analyses of the E. coli mutant Δ arsC (in WC3110 strain). This strain lacks the bacterial As(V) reductase gene and has an intact As(III) extrusion pump; it thus has increased sensitivity to As(V) but not to As(III) [28] . Our analyses showed that At2g21045-Col-0 expression restored Δ arsC growth in the presence of As(V), whereas expression of an At2g21045-Col-0 mutant form with a Cys 113 -to-Gly 113 substitution was unable to complement the Δ arsC phenotype ( Fig. 2d ). In the presence of As(V), the Δ arsC strain expressing At2g21045-Col-0 showed increased As(III) extrusion, similar to the WC3110 wild-type strain ( Fig. 2e and Supplementary Fig. 6a ). Moreover, plant As(V) content as well As(III)/As(V) ratio were significantly higher in Col plants than in the At2g21045 T-DNA mutant ( Fig. 2f and Supplementary Fig. 6b ). Furthermore, ATQ1 purified protein expressed in E. coli exhibited arsenate reductase activity in vitro ( Fig. 2g ) and kinetic parameter ( K m ) for As(V) was in the range of other eukaryotic arsenate reductases previously identified [12] , [28] ( Fig. 2h ). We thus concluded that At2g21045 encodes an As(V) reductase, which we termed Arabidopsis thaliana arsenate reductase QTL1 ( AtARQ1 ). AtARQ1 natural alleles define two frequent haplogroups To test the functional basis of AtARQ1 / At2g21045 natural variation, we analyzed the nucleotide diversity of its coding region in Col-0, Kas-1 and a set of 18 accessions distributed worldwide ( Supplementary Fig. 7a ). We found five missense mutations and two compensatory indels of one and five nucleotides differing between Col-0 and Kas-1, which alter the amino acids in positions 2–19 ( Fig. 3a ). A functional effect of this structural variation in this reductase was supported by the folding disruption predicted by AtARQ1-Kas-1 protein modelling ( Fig. 3b ). Col-0 and Kas-1 define two major haplotypes, as detected by cluster analysis, differentiated by the seven structural polymorphisms described above, as well as 23 silent (synonymous and intronic) mutations ( Supplementary Fig. 7b ). Haplotype network analysis of 827 AtARQ1 sequences from the 1001 Arabidopsis Genome Project ( http://www.1001genomes.org ) showed that Col-0 and Kas-1 haplogroups differ from the A. lyrata branch by one and three of the missense mutations, respectively ( Fig. 3c ). The Col-0 As(V)-tolerant haplogroup thus appeared to be closer to the ancestral allele. Both haplogroups are distributed worldwide, although Kas-1 haplogroup is found at high frequency in Asia ( Supplementary Fig. 7c ). This geographical pattern appears to be determined at least in part by A. thaliana demographic history, as Kas-1 haplogroup distribution overlaps markedly with the Asian-dominant genetic group detected by genome-wide neutral single-nucleotide polymorphism [29] . 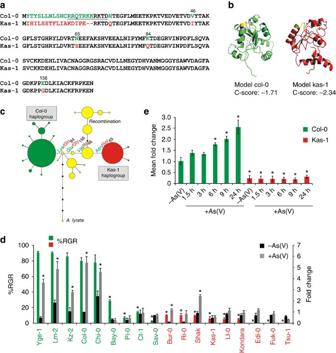Figure 3: Allelic variation atAtARQ1involves structural and regulatory polymorphisms. (a) Alignment of AtARQ1 proteins from Col-0 and Kas-1. Changes in amino acid sequence between Col-0 (green) and Kas-1 (red). Numbers indicate positions of changes. Nuclei localization signal is underlined. (b) Three-dimensional structural models of AtARQ1 proteins from Col-0 and Kas-1 predicted by I-TASSER. Predicted confidence (C-score) rankings are shown.113CX4R118motifs are in yellow. (c) Haplotype network analysis using AtARQ1 proteins from the 1001 Arabidopsis Genome Project andArabidopsis lyrata. Each line segment corresponds to an amino acid substitution. Areas of circles are proportional to frequency and colors depict the two major haplogroups. (d) Northern blot quantification ofAtARQ1expression and %RGR in several Arabidopsis accessions. Plants were grown alone or exposed to 30 μM As(V) 24 h. Bars show mean±s.d. (n=2). %RGR was determined in 18 Arabidopsis accessions representing Col-0 (green) and Kas-1 (red) haplogroups. Bars show mean±s.d. (n=3). (e) Quantitative reverse transcription–PCR time-course analysis ofAtARQ1expression in response to As(V). Col-0 (green) and Kas-1 (red) plants were exposed to 30 μM As(V) for the indicated time. Bars show mean±s.d. (n=3). *P<0.05 Student'st-test. Figure 3: Allelic variation at AtARQ1 involves structural and regulatory polymorphisms. ( a ) Alignment of AtARQ1 proteins from Col-0 and Kas-1. Changes in amino acid sequence between Col-0 (green) and Kas-1 (red). Numbers indicate positions of changes. Nuclei localization signal is underlined. ( b ) Three-dimensional structural models of AtARQ1 proteins from Col-0 and Kas-1 predicted by I-TASSER. Predicted confidence ( C -score) rankings are shown. 113 CX 4 R 118 motifs are in yellow. ( c ) Haplotype network analysis using AtARQ1 proteins from the 1001 Arabidopsis Genome Project and Arabidopsis lyrata . Each line segment corresponds to an amino acid substitution. Areas of circles are proportional to frequency and colors depict the two major haplogroups. ( d ) Northern blot quantification of AtARQ1 expression and %RGR in several Arabidopsis accessions. Plants were grown alone or exposed to 30 μM As(V) 24 h. Bars show mean±s.d. ( n =2). %RGR was determined in 18 Arabidopsis accessions representing Col-0 (green) and Kas-1 (red) haplogroups. Bars show mean±s.d. ( n =3). ( e ) Quantitative reverse transcription–PCR time-course analysis of AtARQ1 expression in response to As(V). Col-0 (green) and Kas-1 (red) plants were exposed to 30 μM As(V) for the indicated time. Bars show mean±s.d. ( n =3). * P <0.05 Student's t -test. Full size image The contribution of AtARQ1 amino acid substitutions to As(V) tolerance variation was evaluated by further analyzing the 18 sequenced accessions. All accessions with the Kas-1 haplotype had an As(V)-sensitive phenotype (RGR<30%), indicating that the Col-0 haplotype is needed for As(V) tolerance ( Fig. 3d , Supplementary Data 1 ). AtARQ1-GFP fusion protein localized in cytoplasm and also in nuclei ( Supplementary Fig. 8a ). AtARQ1 nuclei localization mirrors the localization pattern of cell cycle CDC25 phosphatases [30] that are homologous to arsenate reductases. Accordingly, a predicted nuclear localization signal is present at the N-terminal region of AtARQ1 ( Fig. 3a ). Gene expression analysis showed that As(V) induces AtARQ1 in Col-0 mainly in roots ( Supplementary Fig. 8b ). In contrast Kas-1 has much lower gene expression ( Fig. 3e ). Expression analyses of the 18 accessions confirmed that both haplogroups also differ in AtARQ1 regulation, since Col-0 haplotype accessions showed higher AtARQ1 expression on average than Kas-1 genotypes ( Fig. 3d ). Four Col-0 haplotype accessions nonetheless showed low AtARQ1 expression (Bay-0, Pi-0, Ct-1, Sav-0) and all had an As(V)-sensitive phenotype. These data indicate that both structural and regulatory (cis and/or trans) allelic variations affect AtARQ1 function and thus, As(V) tolerance. One Kas-1 haplotype accession (Shak) showed high AtARQ1 expression but an As(V)-sensitive phenotype ( Fig. 3d ), further supporting the idea that AtARQ1 structural polymorphisms are a major functional cause of natural variation in As(V) tolerance. Non-additive intra-allelic mutations explain ATQ1 function To demonstrate the functional effects of AtARQ1 structural variation, we used complementation of Δ arsC mutant strains with various chimeric AtARQ1 proteins generated by directed mutagenesis ( Fig. 4a ). In bacteria expressing AtARQ1 from Col-0 or Kas-1, these proteins differed greatly in their As(V) reductase activity; Col-0 but not Kas-1 was able to restore bacterial growth and As(III) extrusion ( Fig. 2d,e ). We used Kas-1 sequences to replace the first 23 amino acids after the first methionine ( Fig. 4a ), or single residues at positions 46, 65, 84 or 156 in five Col-0 proteins; these chimeric proteins complemented bacterial growth similar to the Col-expressing bacteria ( Fig. 4b ). This result suggested that several structural changes are necessary to explain functional differences between Col-0 and Kas-1 AtARQ1. This was demonstrated by Δ arsC complementation analysis of AtARQ1-Col-0 proteins with double or triple combinations of the four missense mutations that distinguish Kas-1 from Col-0 haplogroups in network analysis ( Figs 3c and 4a ). These analyses showed that expression of AtARQ1 bearing any combination of the three missense mutations that differentiate Kas-1 from A. lyrata (positions 156, 46 and 65; Fig. 3c ) does not restore Δ arsC As(V) sensitivity ( Fig. 4b ). Bacteria transformed with AtARQ1 bearing Kas-1 mutations at positions 65/84 had an As(V)-resistant phenotype comparable to that of the wild-type strain ( Fig. 4b ), which implies that the Lys 84 /Gln 84 missense mutation does not affect protein function, and suggests that A. lyrata AtARQ1 encodes a functional As(V) reductase. At difference from most plant QTL identified so far, which are due to single functional polymorphisms [31] , natural variation at AtARQ1 involves several structural nucleotide polymorphisms that act in a non-additive manner on As(V) reductase function. Recent studies showed the first large effect natural alleles from plants due to multiple additive functional polymorphisms [32] , [33] . Our results provide evidence of the higher complexity that can underlie natural alleles and the combinatorial impact of multiple intra-allelic mutations with little or no additive effect, in the generation of large effect alleles that contribute to quantitative variation and evolution in plants [34] . It is very unlikely that the AtARQ1 -Kas-1 allele is null, since a fully expressed protein is predicted. Although the true functional features of AtARQ1 variation are unknown, our findings suggest that several functional allelic polymorphisms have contributed to its maintenance in nature. 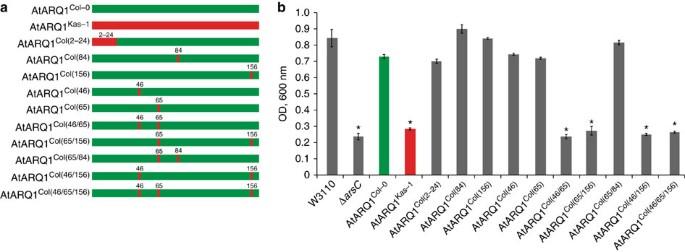Figure 4: Several structural non-additive polymorphisms affect AtARQ1 function. (a) Diagram of AtARQ1 from Col-0, Kas-1 and their chimeric proteins. Numbers indicate positions at which the Kas-1 amino acid was introduced into the Col-0 protein. (b) Complementation analysis ofE. coliΔarsCmutant overexpressing different chimeric AtARQ1 proteins indicated ina. All strains were grown in 1 mM As(V). Bars show mean±s.d. (n=3). *P<0.001 (Student’st-test). Figure 4: Several structural non-additive polymorphisms affect AtARQ1 function. ( a ) Diagram of AtARQ1 from Col-0, Kas-1 and their chimeric proteins. Numbers indicate positions at which the Kas-1 amino acid was introduced into the Col-0 protein. ( b ) Complementation analysis of E. coli Δ arsC mutant overexpressing different chimeric AtARQ1 proteins indicated in a . All strains were grown in 1 mM As(V). Bars show mean±s.d. ( n =3). * P <0.001 (Student’s t -test). Full size image This study shows the use of natural variation to detect alleles involved in plant adaptation to environmental chemical stress. Identification of AtARQ1 demonstrates the critical role of a new group of As(V) reductases in As(V) tolerance and detoxification in plants. This role coincides with the enhanced As(V) reductase activity observed in naturally selected As(V) hyper-accumulator plants, which triggers an increase in plant capacity to detoxify As(III) [35] . To date, the mechanism of this enhanced activity was not known. The identification of several AtARQ1 functional polymorphisms further indicates considerable complexity in the natural variation and evolution of As(V) secondary metabolism genes with pleiotropic effect on a trait related to fitness, such as As(V) tolerance. Thus, AtARQ1 provides an additional molecular component for understanding plant adaptation to arsenate. Furthermore, since AtARQ1 gene contributes to A. thaliana natural variation for arsenate tolerance at organism level, it shows a higher potential for phytoremediation than other genes involved in arsenic metabolism whose modifications are not maintained in nature. Plant materials and growth conditions A collection of 82 Arabidopsis thaliana accessions with worldwide distribution was analyzed for As(V) tolerance ( Supplementary Data 1 ). Two RIL populations of 93 and 150 lines derived from the crosses Col gl-1 x Kas-1 (ref. 18 ) and Col-0 x Tsu-0 (ref. 36 ), respectively, were used for QTL mapping for As(V) tolerance as estimated by the RGR assay ( Supplementary Data 2,3 ). The At2g21045 T-DNA mutant (GK-868F11) that bears an insertion in the second exon was obtained from the GABI-Kat [37] . Homozygous knockout plants were selected by PCR using the T-DNA-specific primer 5′-ATAATAACGCTGCGGACATCTACATTTT-3′ and the At2g21045-specific primer 5′-AAATGTTCATCTTTCTTGCAAACC-3′. The At5g03455 T-DNA mutant (GK-772G06) [37] with an insertion in AtACR2 and its overexpression line were used. Both lines were kindly provided by Professor Francis Dennis, Cardiff University (Wales, UK). Seedlings were grown on Johnson medium supplemented with Pi (KH 2 PO 4 ) at various concentrations, depending on the experiment; 1 mM Pi was used for complete medium (+Pi), and 5 μM for phosphate-starvation medium (−Pi). In general, for As(V) treatment (NaH 2 AsO 4 ·7H 2 O), plants were grown on Johnson medium +Pi for 7 days, transferred to −Pi medium for 2 days, and finally to liquid −Pi medium alone or supplemented with 30 μM As(V). For all molecular and biochemical analyses, Arabidopsis plants were grown in a culture chamber in a 16-h light/8-h dark regime (24 °C/21 °C). QTL analyses for As(V) tolerance For QTL mapping, the 93 or 150 RILs of the Col gl-1 x Kas-1 or Col-0 x Tsu-0 populations, respectively, were grown and phenotyped using the RGR assay described in physiological section. All lines from each population were grown simultaneously in the same growth chamber, at 21 °C and long day photoperiod (16-h light/8-h dark regime) organized in a two complete blocks design. Each block contained 13–30 plants per RIL grown in a single vertical plate. For each RIL, the mean percentage of plants that showed %RGR was calculated from the two blocks, and means were transformed by the angular transformation (arcsin √). These data were analyzed for QTL mapping of As(V) using the genetic map with 99 and 79 markers previously developed for the Col gl-1 x Kas-1 and Col-0 x Tsu-0 populations [18] , [36] . QTL were mapped by the multiple QTL mapping method implemented in MapQTL v.4.0 software [38] . QTL were detected using LOD thresholds of 3, corresponding to an approximate genome-wide significance α =0.01, as estimated with the MapQTL permutation test. The additive allele effect and the percentage of variance explained by each QTL, as well as the total variance explained by the additive effects of all QTL detected for the trait analyzed, were obtained from multiple QTL mapping method models. Development of NIL and fine mapping of ATQ1 NIL bearing ATQ1 -Kas-1 alleles in Col gl-1 background were developed from the selected RIL CK-893. The genetic background of this RIL was Col gl-1 except for the complete chromosome 2 (where ATQ1 is located) and four genomic regions of chromosomes 1 and 5. CK-893 was backcrossed to Col gl-1 and an F 2 population of 600 plants was analyzed for 18 indel, simple sequence length polymorphism and the morphological ( gl-1 ) marker (see Supplementary Data 4 ) to select Kas-1 homozygous individuals for the introgression fragment around ATQ1 and Col gl-1 for the remaining genomic segments. From this analysis, we obtained four F 2 individuals homozygous for all but one of the regions. F 3 and F 4 plants were analyzed to obtain the four final NILs (128, 154, 155 and 248) with a single Kas-1 introgression fragment of ~12 Mb on the Col gl-1 background. The NIL128 and 155 Kas-1 introgression fragments are located between physical positions 7 and 19.6 Mb, which overlap the NIL154 and 248 ATQ1 introgressed region located between positions 0 and 11.1 Mb ( Supplementary Fig. 1d ). To characterize ATQ1 , the NILs, parental lines and F 1 plants derived from crosses of Col gl-1 × NIL128 were grown simultaneously as described for RIL populations. Fine mapping of ATQ1 was carried out using an F 2 mapping population of 679 plants derived from a cross between NIL128 and Col. These plants were genotyped with 11 indel and simple sequence length polymorphism markers around the ATQ1 region between physical positions 7 and 11.1 Mb ( Supplementary Fig. 3 ). ATQ1 was genotyped in the QTL region by analyzing the As(V) tolerance phenotype of F 3 families derived from selected F 2 recombinant plants. To confirm and validate the fine mapping results from F 3 families, we obtained a set of 16 F 4 homozygous NIL with partially overlapping introgression fragments from selected recombinants [39] . Sister plants (16–20) from selected F 3 families were genotyped around the ATQ1 region, and homozygous recombinant individuals were selected and selfed. One of the F 4 offspring from the selected F 3 individual was again genotyped with markers flanking the recombination point to confirm the genotype of the final homozygous recombinant NIL. Physiological measurements For As(V) tolerance analysis, plants were grown on Johnson medium in Pi starvation conditions (−Pi) for 7 days and transferred to 15 μM As(V) alone or with 1 mM TNBS for 1 day; plants were then grown in 1 mM Pi (+Pi) plates in a vertical position for 1 day. The percentage of plants that showed %RGR was then determined. Alternatively, plants were grown on Johnson Pi medium alone or with various As(V) concentrations (7 days). Main root length was measured using ImageJ v.1.48c (ref. 40 ). For arsenic accumulation experiments, plants were grown on plates with half-strength Bates and Lynch medium solidified with 0.4% bacto-agar with 30 μM Pi, covered with 0.4-mm pore nylon mesh. Seeds were sown onto the mesh and cultured for 7 days. Plants were treated with PI and PII buffers [41] . Arsenic accumulation and uptake experiments were performed in 50 ml pots using 5 μM As(V), for 24 h and 1 h, respectively. Plants were dried (60 °C, 5 days), mineralized with HNO 3 –H 2 O 2 in a pressure digester, and analyzed for total arsenic content by inductively coupled plasma-mass spectrometry. Complementation of bacteria Escherichia coli strains W3110 (wild type; K12 F2 IN (rrnD-rrnE)) [42] and WC3110 (Δ arsC ) (Δ arsC ; W3110Δ arsC ::Kan) [28] alone or transformed with the AtARQ1 constructs encoding different versions of the protein were used for As(V) sensitivity assays. Three replicates of the Δ arsC strain bearing AtARQ1 variants were grown in liquid LB medium with shaking (37 °C, overnight). The OD 600 nm was measured, cultures were diluted with low Pi medium [39] to OD 600 nm =0.2, and allowed to grow alone or in various As(V) concentrations (30 °C, 24 h). Bacterial growth in different As(V) concentrations was determined at OD 600 nm . Expression and purification of AtARQ1 A culture of E. coli BL21 cells, harbouring the plasmid pDEST17- AtARQ1 , was grown in LB medium containing 100 μg ml −1 of ampicillin at 37 °C until the OD600 nm was 0.6. Isopropyl-β- D -thiogalactopyranoside was then added to a final concentration of 0.4 mM and growth continued for 3.5 h at 30 °C. Cells were then harvested by centrifugation, frozen in liquid nitrogen and resuspended in 50 mM Tris-HCl buffer (pH 8), 300 mM NaCl (lysis buffer) supplemented with 10 mM imidazole and 1 mM phenylmethylsulfonyl fluoride. After sonication and centrifugation, the supernatant was applied to a Ni-NTA agarose resin (QIAGEN), previously equilibrated with the same buffer, and incubated for 2 h at 4 °C in a rotatory wheel. Subsequently the resin was packed into a column, washed with 10 column volumes of lysis buffer with 10 mM imidazole, and twice with the same buffer containing 20 mM of imidazole. Protein was eluted with increasing concentration of imidazole (from 100 to 500 mM) in lysis buffer. The His-tagged recombinant protein eluted at an imidazole concentration of 100 mM. Protein concentration was estimated in a 12% polyacrylamide gel by comparison with a bovine serum albumin standard. Determination of As(V)-reductase activity The assay reaction mixture contained 50 mM Tris-HCl buffer (pH 7.5), 7 μg of recombinant His-AtARQ1 protein in the presence of the indicated As(V) concentration. The final reaction volume was 200 μl. Reaction was started by the addition of 0.5 mM dithiothreitol and was allowed to proceed for the indicated times at 37°C. Reaction was stopped by the addition of 20 mM mersalyl, to displace thiol-bound As(III), and 15 s later, proteins were precipitated by the addition of 3 volumes of ice-cold methanol and kept at −80 °C until they were analyzed for As(III) quantification. The reactions were centrifuged (5500 g , 10 min) and supernatant was passed through a 22-μm nylon syringe before arsenic speciation using HPLC–ICP–MS as described below. In parallel, reactions containing the complete assay mix without enzyme were performed to quantify non-enzymatic reduction of arsenate. Kinetic parameters were estimated measuring the time course of As(III) production using 6 μg of recombinant His-AtARQ1 with increasing concentrations of arsenate in the assay mix. Non-enzymatic reduction of As(V) was subtracted and data was analyzed using SigmaPlot v.12.5. Arsenic species analysis Arsenic species analyses were performed using plants, bacteria and purified recombinant AtARQ1 protein. Plants were grown and treated as for arsenic accumulation experiments (see above, physiological measurements section), and exposed to 5 μM As(V) in 50 ml pots during 24 h. Plants were dried (60 °C, 5 days) and 20 mg were used as samples for arsenic species quantification. For bacteria, different E. coli strains were grown in liquid LB medium with shaking (37 °C, overnight). OD 600 nm was measured, all cultures were diluted with low Pi medium [43] to OD 600 nm =0.2 and allowed to grow, alone or with 1 mM As(V) (30 °C, 24 h). Since most As(III) is extruded in bacteria, cultures were centrifuged and 1 ml of supernatant was collected. Lyophilized supernatant (20 mg) was used as cell-free extract for arsenic species quantification. Arsenic species from plant and bacterial samples were extracted with (1:1) methanol:water using an ultrasonic homogenizer SONOPLUS HD 2200 (30%, 60 s). Extracts were centrifuged (5500 g , 10 min) and supernatant was passed through a 22-μm nylon syringe before injection in the HPLC for arsenic speciation. Diluted samples were injected onto an anion-exchange column PRP-X100 (250 mm × 4.1 mm, particle size 10 μm; Hamilton, Reno, NV, USA). Arsenic species were eluted in 10 mM HPO 4 −2 /H 2 PO 4 −1 , 2% (v/v) MeOH mobile phase, at a 1.5 ml min −1 flow rate. To test the efficiency of the applied method, three replicates of the extracts were individually digested with HNO 3 –H 2 O 2 to compare the total arsenic content (ICP–MS) with the concentration sum of all arsenic species (LC–ICP–MS) in the initial extracts. As(III) was quantified on an As(III) calibration curve; As(V) in the sample was used as an internal normalization standard. Analytical quality control used for total arsenic content and arsenic species was validated by analyzing several Certified Reference Material (reference number SRM 1568a; NIST, USA and CRM-627; BCR, Belgium). Good agreement was found for both reference materials tested (<10% uncertainty considering 95% confidence level). Extraction recovery was performed by spiking the samples with known amounts of different arsenic species obtaining recoveries between 80–100%. Binary construct and plant transformation To generate At2g21045-overexpressing lines, the full-size coding region of the Col-0 At2g21045 gene was amplified with primers At2g21045Fp/At2g21045Rp ( Supplementary Data 5 ), cloned into the pENTR/D-TOPO vector (Invitrogen), and inserted into the pGWB2 (ref. 44 ) binary vector containing the constitutive 35S promoter, using the LR recombination reaction (Invitrogen). This binary construct was introduced into Agrobacterium tumefaciens strain C58C1 and transformed in NIL128 plants using the floral dip transformation method [45] . Transformants were selected on 40 mg l −1 hygromycin-containing medium. Bacterial constructs For bacterial complementation, full-size At2g21045 complementary DNA (cDNA) from Col-0 and Kas-1 were amplified with primers At2g21045F/At2g21045R and At2g21045kF/At2g21045R, respectively ( Supplementary Data 5 ). The products were excised with BamHI and HindIII and cloned into the pET-23a vector (Novagen) bearing the T7 promoter. Using At2g21045 cDNA (Col-0) as template, we generated 10 versions of At2g21045 cDNA by PCR site-directed mutagenesis to introduce Kas-1 single-nucleotide polymorphism (primers listed in Supplementary Data 5 ). All protein versions were cloned into the pET-23a vector (Novagen) in the BamHI and HindIII sites. All constructs were transformed in the E. coli strain WC3110 (Δ arsC ) (Δ arsC ; W3110Δ arsC ::Kan) [28] . Subcellular localization Full length AtARQ1 cDNA was cloned into pGWB5 plasmid [44] , to obtain AtARQ1-GFP fusion protein. N. benthamiana leaves were transiently transformed by agroinfiltration with this construct and with the P19 suppressor of silencing (1:1) as described [46] . Subcellular localization was observed in epidermal cells 72 h post agroinfiltration, using a Bio-Rad Radiance 2100 laser scanning confocal imaging system with LaserSharp2000 version 5.2 imaging software. Green fluorescent protein fluorescence was excited at 488 nm using an argon ion laser and subsequently passed through a 515/30-nm emission filter excluding chlorophyll autofluorescence. Expression analyses RNA was extracted with RNAwiz reagent (Ambion). For Northern blot, 15 μg total RNA was loaded in each lane. For RNA electrophoresis, transfer to nylon membranes and hybridization was done using standard procedures [47] . The probe was amplified by PCR using primers At2g21045kF-46/At2g21045Rp ( Supplementary Data 5 ) and labelled with T4 polynucleotide kinase (Roche) and 50 μCi γ- 32 P-ATP. Films were scanned and blot signal intensity quantified with ImageJ v.1.48c (ref. 40 ). To analyze AtARQ1 expression, we divided normalized AtARQ1 intensity in each accession by that in Col-0. Quantitative reverse transcription–PCR was performed on three independent biological samples as described [48] . Each sample was normalized using EF1α (for primer pairs, see Supplementary Data 5 ). Sequence analyses A 1.3-kb genomic fragment of AtARQ1 (from ATG to 3′UTR) was sequenced in Kas-1 and 18 accessions using an ABI PRISM 3700 DNA analyzer. DNA and protein sequences were aligned with Clustal Omega ( http://www.ebi.ac.uk/Tools ) and alignments were inspected and edited by hand. The percentages of amino acid sequence identity (%ID) and similarity between AT2G21045 and the other proteins in the alignment was calculated using CLUSTALW. A haplotype network of AtARQ1 was constructed from protein sequences of 827 accessions from the Arabidopsis 1001 Genomes Project ( http://www.1001genomes.org ) using NETWORK v.4.5 ( http://www.fluxus-engineering.com ) with the median-joining method. The first 24 amino acids of AtARQ1 were not included in these analyses, as they contain the two compensatory indel and have a higher sequencing error rate [29] . Molecular modelling The three-dimensional structure of AT2G21045 was modelled using I-TASSER [49] ( http://zhanglab.ccmb.med.umich.edu/I-TASSER ). Models were built mainly on the NMR solution structure of A. thaliana protein AT5G66040 (PDB ID 1TQ1, chain A), ranked as the best template by 6 of the 10 threading programs in I-TASSER. At5g66040 was determined to have the most similar structure to AT2G21045 by TM-ALIGN [50] . All models were inspected visually and images were rendered using Pymol v1.4.1. A scoring function (C-score) based on the relative clustering structural density and consensus significance score of multiple threading templates was introduced to estimate the accuracy of I-TASSER predictions. Accession codes: Sequence data for the ATQ1 gene of 19 wild accessions have been deposited in GenBank/EMBL/DDBJ under the accession codes KF938555 to KF938573 . How to cite this article: Sánchez-Bermejo, E. et al. Natural variation in arsenate tolerance identifies an arsenate reductase in Arabidopsis thaliana . Nat. Commun. 5:4617 doi: 10.1038/ncomms5617 (2014).